FBH1 co-operates with MUS81 in inducing DNA double-strand breaks and cell death following replication stress The molecular events occurring following the disruption of DNA replication forks are poorly characterized, despite extensive use of replication inhibitors such as hydroxyurea in the treatment of malignancies. Here, we identify a key role for the FBH1 helicase in mediating DNA double-strand break formation following replication inhibition. We show that FBH1-deficient cells are resistant to killing by hydroxyurea, and exhibit impaired activation of the pro-apoptotic factor p53, consistent with decreased DNA double-strand break formation. Similar findings were obtained in murine ES cells carrying disrupted alleles of Fbh1. We also show that FBH1 through its helicase activity co-operates with the MUS81 nuclease in promoting the endonucleolytic DNA cleavage following prolonged replication stress. Accordingly, MUS81 and EME1-depleted cells show increased resistance to the cytotoxic effects of replication stress. Our data suggest that FBH1 helicase activity is required to eliminate cells with excessive replication stress through the generation of MUS81-induced DNA double-strand breaks. Faithful chromosome duplication is fundamental for the maintenance of genome stability and cell proliferation. However, cellular DNA is particularly vulnerable to incurring damage during the replication process. Even in the absence of exogenously inflicted stress, DNA replication forks may encounter a large number of potentially damaging adducts or lesions in the template DNA in each cell cycle. Undetected or inappropriately repaired lesions can lead to irreversible changes to chromosome structure, which can promote genomic instability and potentially the development of cancer [1] , [2] . To ensure the fidelity of DNA replication, cellular mechanisms have evolved to detect any perturbation of replication fork progress, and ensure that replication errors are corrected before cell division occurs. If the lesions cannot be corrected in a timely fashion, cells are eliminated through cell death pathways [1] , [2] , [3] . Replication perturbation can lead to fork stalling, and in case of widespread stalling of replication forks cells enter a state commonly referred to as ‘replicative stress’ [1] . If these stress-activating obstacles are not removed or circumvented, forks can collapse, a poorly understood process where the replication machinery dissociates from the DNA and DNA double-strand breaks (DSBs) are subsequently generated [1] . Recent data suggest that oncogene activation can stress replication forks to such an extent that additional genetic lesions arise, leading to further progression of tumorigenesis [4] . Nevertheless, this feature of cancer cells can also be an ‘Achilles’ heel’, because neoplastically transformed cells experience enhanced levels of constitutive, oncogene-induced replication stress [4] . Hence, cancer cells potentially can be eliminated by an acute overload of replication stress, through treatment with commonly used anti-cancer drugs that disturb replication forks, such as hydroxyurea (HU), gemcitabine and cytosine arabinoside. HU blocks DNA synthesis by depleting the cellular pool of deoxyribonucleotides (dNTPs) through inhibition of ribonucleotide reductase, the enzyme that converts NTPs into dNTPs. Cells experiencing replication stress activate checkpoint pathways, which in budding yeast have been shown to stabilize stalled replication forks [1] , [5] . In general, much less is known about the processing of stalled replication forks in mammalian cells. Following prolonged replication arrest, the disassembly of the replication machinery can be accompanied by the cleavage of the fork by the structure-specific endonuclease MUS81 (ref. 6 ). This generates a one-ended DSB that is thought to be the precursor for recombination-dependent replication fork restart [7] , [8] . However, the processes that promote fork collapse and lead to the generation of a substrate for MUS81 are currently unknown. The helicase FBH1 has been shown to participate in the cellular response to replication stress, and is known to localize to sites of stalled replication forks [9] . FBH1 is a member of the evolutionary conserved UvrD family of DNA helicases [10] . Mammalian FBH1 protein has, like other UvrD helicases, been shown to possess 3′–5′ DNA helicase activity [10] . Analysis of the biochemical properties of the protein suggested a number of potential cellular substrates including replication forks [10] . Other members of the UvrD family, including E. coli UvrD itself and S. cerevisiae Srs2 protein, have been implicated in the processing of stalled replication forks and in regulating homologous recombination (HR) [11] . However, S. cerevisiae lacks a true FBH1 ortholog. Although the biological role of FBH1 is unclear, evidence from studies in the fission yeast, S. pombe, indicate that FBH1 operates as a regulator of RAD51 to suppress homologous recombination [12] . However, it is unclear to what extent this is a conserved function, as studies in vertebrate systems have revealed only a minor role for FBH1 in restraining HR [9] , [13] . Here, we have investigated how mammalian FBH1 participates in the response to replication stress. We found that FBH1 has a major role, mediated through its helicase activity, in activating MUS81-dependent cleavage of stalled replication forks. The FBH1-dependent DSBs that arise from prolonged replication arrest induce checkpoint signalling, a p53-dependent response, and ultimately cell death. Accordingly, we found that cells deficient in FBH1 and MUS81 are more resistant to HU. We propose a model whereby FBH1-driven processing of stalled forks promotes MUS81-mediated DNA cleavage to amplify the checkpoint signal and eliminate cells with high levels of replication stress. FBH1 promotes DNA breakage and cell death in response to replication stress Human FBH1 is known to be rapidly recruited to ssDNA regions and it has been suggested to have a role in the processing of stalled replication forks [9] . In order to gain insight into the role of FBH1 in the replication stress response, we generated a human osteosarcoma (U2OS) cell line carrying an FBH1-specific short hairpin RNA (shRNA) expressed from plasmid under the control of a doxycycline inducible promoter. Following induction of the shRNA by doxycycline for 48 h, the cellular pool of the FBH1 protein was depleted ( Fig. 1a ). We then exposed cells to HU for various times, and quantified clonogenic survival. Prolonged treatment with HU is known to cause cell death, most likely because of accumulation of cytotoxic DSB lesions [14] . Strikingly, we found that cells depleted for FBH1 were significantly more resistant to HU treatment compared with non-depleted cells ( Fig. 1b ). In contrast to this, we did not observe any effect of FBH1 status on survival following exposure to ionizing radiation that induces replication-independent DNA breakage (data not shown). To rule out the possibility that the observed phenotype was due to there being fewer cells in S-phase in the depleted cells, we showed that depletion of FBH1 did not affect cell cycle distribution as examined by flow cytometry and EdU incorporation ( Supplementary Fig. S1 ). 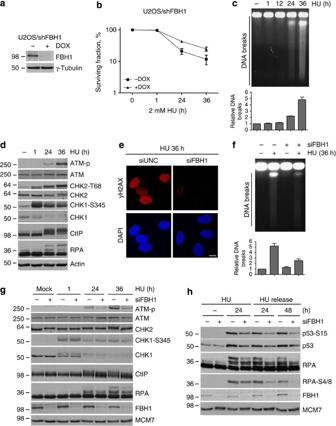Figure 1: FBH1 promotes DNA breakage and cell death in response to replication stress (a) U2OS/shFBH1 cells were either induced or not with doxycycline for 48 h, collected and subjected to immunoblotting with the indicated antibodies. The sizes of molecular mass standards (in kDa) are shown on the left. (b) U2OS/shFBH1 cells were induced or not with doxycycline for 48 h, before treatment with 2 mM HU for the indicated times. Cells were plated and surviving clones were scored 10–12 days later. Graph depicting the surviving fractions is shown. Experiments were done in triplicate and error bars represent s.d. (c) (Top) U2OS cells were treated with 2 mM HU, collected at the indicated timepoints and subjected to PFGE analysis. Bands representing DNA breaks are shown. (Bottom) Experiments were done in triplicate, bands were quantified using ImageJ software and error bars represent s.d. (d) U2OS cells were treated as per panel (c), and were subjected to immunoblotting with the indicated antibodies. (e) U2OS cells were transfected with siRNA targeting FBH1 (pool) or negative control for 48 h before treatment with 2 mM HU for 36 h. Cells were fixed and subjected to immunofluorescence staining with the indicated antibodies. Scale bar, 10 μm. (f). (Top) U2OS cells were transfected with siRNA targeting FBH1 (pool) or negative control for 48 h before treatment with 2 mM HU for 36 h. Cells were collected and subjected to PFGE analysis. Bands representing DNA breaks are shown. (Bottom) Experiments were done in triplicate, bands were quantified using ImageJ software and error bars represent s.d. (g) U2OS cells were transfected with FBH1 (pool) or negative control siRNA for 48 h before treatment with 2 mM HU. Cells were collected at the indicated timepoints and subjected to immunoblotting with the indicated antibodies. (h) U2OS cells were transfected with FBH1 (pool) or negative control siRNA for 48 h before treatment with 2 mM HU for 24 h, before release for the indicated durations. Cells were collected and subjected to immunoblotting with the indicated antibodies. Figure 1: FBH1 promotes DNA breakage and cell death in response to replication stress ( a ) U2OS/shFBH1 cells were either induced or not with doxycycline for 48 h, collected and subjected to immunoblotting with the indicated antibodies. The sizes of molecular mass standards (in kDa) are shown on the left. ( b ) U2OS/shFBH1 cells were induced or not with doxycycline for 48 h, before treatment with 2 mM HU for the indicated times. Cells were plated and surviving clones were scored 10–12 days later. Graph depicting the surviving fractions is shown. Experiments were done in triplicate and error bars represent s.d. ( c ) (Top) U2OS cells were treated with 2 mM HU, collected at the indicated timepoints and subjected to PFGE analysis. Bands representing DNA breaks are shown. (Bottom) Experiments were done in triplicate, bands were quantified using ImageJ software and error bars represent s.d. ( d ) U2OS cells were treated as per panel ( c ), and were subjected to immunoblotting with the indicated antibodies. ( e ) U2OS cells were transfected with siRNA targeting FBH1 (pool) or negative control for 48 h before treatment with 2 mM HU for 36 h. Cells were fixed and subjected to immunofluorescence staining with the indicated antibodies. Scale bar, 10 μm. ( f ). (Top) U2OS cells were transfected with siRNA targeting FBH1 (pool) or negative control for 48 h before treatment with 2 mM HU for 36 h. Cells were collected and subjected to PFGE analysis. Bands representing DNA breaks are shown. (Bottom) Experiments were done in triplicate, bands were quantified using ImageJ software and error bars represent s.d. ( g ) U2OS cells were transfected with FBH1 (pool) or negative control siRNA for 48 h before treatment with 2 mM HU. Cells were collected at the indicated timepoints and subjected to immunoblotting with the indicated antibodies. ( h ) U2OS cells were transfected with FBH1 (pool) or negative control siRNA for 48 h before treatment with 2 mM HU for 24 h, before release for the indicated durations. Cells were collected and subjected to immunoblotting with the indicated antibodies. Full size image To corroborate the above findings, we examined DNA damage accumulation after HU treatment. We found that DNA DSB formation was evident after treatment for 24 h as evidenced by pulsed-field gel electrophoresis (PFGE) that detects DNA breaks ( Fig. 1c ), a finding that is in agreement with a number of previous studies [6] , [15] . Furthermore, treatment with HU led to checkpoint activation at the time of DNA DSB accumulation, including robust ATM activation and the phosphorylation of key downstream targets like CtIP and CHK2 ( Fig. 1d ) [16] , [17] . As DNA breaks induced by prolonged HU treatment promote cell death, we addressed if FBH1 was involved in mediating this cytotoxic DNA breakage. Using the phosphorylation of the DNA damage marker, H2AX (γH2AX) in immunofluorescence staining, we found that cells depleted for FBH1 using small interfering RNA (siRNA) ( Supplementary Fig. S1 ), accumulated substantially lower amounts of this marker following prolonged treatment with HU, suggesting a lower abundance of DNA breaks ( Fig. 1e ). Although γH2AX is widely used as a marker of DNA damage it has been shown also to be phosphorylated by ATR in a DSB-independent manner [18] . In order to address if the decreased γH2AX observed in FBH1-depleted cells was in fact due to decreased DNA breakage we used PFGE, which detects breaks directly. Using PFGE, we found that cells depleted for FBH1, using both sh- and siRNA showed a dramatic reduction in DNA breakage compared with non-depleted cells, following HU treatment ( Fig. 1f and Supplementary Fig. S1 ). These data are in agreement with the higher level of clonogenic survival observed in FBH1-depleted cells. The loss of FBH1 also reduced ATM-dependent DSB signalling events (phosphorylation of CHK2 and CtIP), as well as the DNA-PK dependent phosphorylation of RPA in response to replication stress ( Fig. 1g ), consistent with reduced DNA DSB formation. During recovery from HU treatment, DNA repair pathways are invoked to seal the DNA breaks, and hence allow cell cycle progression to be resumed. At the same time, checkpoints become deactivated in line with the DNA being repaired [19] . In the case of overwhelming or irreparable amounts of DNA damage, cells undergo apoptosis. To examine how FBH1-depleted cells recovered from replication arrest, we applied HU for 24 h and then released cells from the block. We found that cells depleted for FBH1 showed a rapid decrease in the magnitude of the checkpoint signalling response as well as decreased expression and activation of the pro-apoptotic tumour suppressor p53 ( Fig. 1h and Supplementary Fig. S1 ), indicating a lower abundance of DNA breaks as compared with non-depleted cells. The phospho-RPA and phospho-p53 that had emerged in FBH1-depleted cells during HU exposure rapidly became dephosphorylated after HU release. Taken together, these data suggest that prolonged HU treatment induces DNA breaks in S-phase in an FBH1-dependent manner. In parallel, we also addressed whether FBH1 ablation might affect fork restart after replication stress, which could affect clonogenic survival. However, using the DNA fibre assay we did not find evidence for a role of FBH1 in this process ( Supplementary Fig. S1 ). FBH1 helicase activity promotes DNA DSB formation Next, we assessed the contribution of the helicase activity of FBH1 to the checkpoint signalling seen following replication arrest. As ablation of FBH1 led to strong reduction in DNA breakage following HU treatment, we speculated that ectopic expression of FBH1 might have the opposite effect and potentiate the HU response by inducing more breakage. We found that expression of wild-type FBH1 significantly sensitized cells to HU treatment, as measured by clonogenic survival assays ( Fig. 2a ). Importantly, helicase-deficient FBH1 did not sensitize cells to HU suggesting that FBH1 helicase activity mediates the response to HU treatment. FBH1 expression in the absence of HU did not significantly affect survival, implying that FBH1 functions predominantly in the response to replication stress. This is also consistent with previous findings that FBH1 is only localized to sites of replication stress and not to replication forks per se [9] . The expression levels of wild-type and helicase-dead FBH1 alleles were comparable, ruling out differential expression as cause of the observed phenotypes ( Fig. 2b ). Following treatment with HU, we found that expression of wild-type, but not a helicase-dead version of FBH1 led to marked ATM phosphorylation, as well as pronounced phosphorylations of its target proteins CHK2, CtIP and p53 in response to HU treatment ( Fig. 2b and Supplementary Fig. S1F ). This indicates that FBH1 promotes checkpoint signalling through a helicase-dependent generation of DNA DSBs. Moreover, we also observed a strong FBH1 helicase-dependent generation of DNA breaks in cells exposed to HU ( Fig. 2c ). The increased breakage observed upon exposure to HU in FBH1 wild-type, but not helicase dead, expressing cells, were accompanied by increased levels of γH2AX as seen by immunofluorescence ( Fig. 2d ). 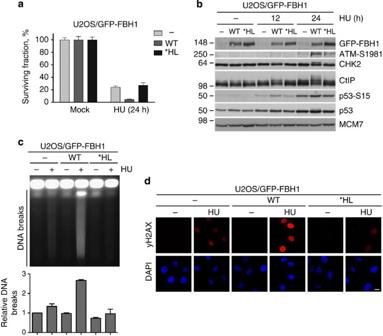Figure 2: FBH1 helicase activity drives DNA DSB formation after replication stress (a) U2OS cells expressing either wild-type (WT) or helicase mutant (*HL) GFP-tagged FBH1 in a doxycycline inducible fashion were either induced or not with doxycycline for 24 h before treatment with 2 mM HU for 24 h. Cells were plated and surviving clones were scored 10–12 days later. Graph depicting the surviving fractions is shown. Experiments were done in triplicate and error bars represent s.d. (b) U2OS/GFP-FBH1 WT or *HL cell lines were induced or not with doxycycline for 24 h before treatment with 2 mM HU for 12 or 24 h. Cells were collected and subjected to immunoblotting with the indicated antibodies. The sizes of molecular mass standards (in kDa) are shown on the left. (c) (Top) U2OS/GFP-FBH1 WT or *HL cell lines were induced or not with doxycycline for 24 h before treatment with 2 mM HU for 24 h. Cells were collected and subjected to PFGE analysis. Bands representing DNA breaks are shown. (Bottom) Experiments were done in triplicates, bands were quantified using ImageJ software and error bars represent s.d. (d) U2OS/GFP-FBH1 WT or *HL cell lines were induced or not with doxycycline for 24 h before treatment with 2 mM HU for 24 h. Cells were fixed and subjected to immunofluorescence staining with the indicated antibodies. Scale bar, 10 μm. Figure 2: FBH1 helicase activity drives DNA DSB formation after replication stress ( a ) U2OS cells expressing either wild-type (WT) or helicase mutant (*HL) GFP-tagged FBH1 in a doxycycline inducible fashion were either induced or not with doxycycline for 24 h before treatment with 2 mM HU for 24 h. Cells were plated and surviving clones were scored 10–12 days later. Graph depicting the surviving fractions is shown. Experiments were done in triplicate and error bars represent s.d. ( b ) U2OS/GFP-FBH1 WT or *HL cell lines were induced or not with doxycycline for 24 h before treatment with 2 mM HU for 12 or 24 h. Cells were collected and subjected to immunoblotting with the indicated antibodies. The sizes of molecular mass standards (in kDa) are shown on the left. ( c ) (Top) U2OS/GFP-FBH1 WT or *HL cell lines were induced or not with doxycycline for 24 h before treatment with 2 mM HU for 24 h. Cells were collected and subjected to PFGE analysis. Bands representing DNA breaks are shown. (Bottom) Experiments were done in triplicates, bands were quantified using ImageJ software and error bars represent s.d. ( d ) U2OS/GFP-FBH1 WT or *HL cell lines were induced or not with doxycycline for 24 h before treatment with 2 mM HU for 24 h. Cells were fixed and subjected to immunofluorescence staining with the indicated antibodies. Scale bar, 10 μm. Full size image Murine ES cells devoid of Fbh1 helicase activity are resistant to replication stress As the above data were all generated using si- and shRNA-treated cells, we sought an alternative system in which to substantiate our findings. To do this we generated mouse embryonic stem (MES) cells carrying bi-allelic deletions in the FBH1 helicase domain ( Supplementary Fig. S2 ). Southern blotting and western blotting analysis confirmed the removal of the alleles/full-length FBH1 protein ( Fig. 3a . RT–PCR was performed to monitor expression of the targeted alleles ( Supplementary Fig. S2 ). Notably, wild-type and the helicase-null MES cells had equivalent DNA replication profiles ( Supplementary Fig. S2 ). We then evaluated the response of these cells to HU, and we found that the helicase-null MES cells were also more resistant to HU treatment compared with wild-type cells ( Fig. 3c ). Interestingly, this effect was not only observed in response to HU, but also following treatment with the DNA polymerase inhibitor aphidicolin ( Fig. 3c ), suggesting that FBH1 generally responds to replication stress, and not to nucleotide depletion specifically. As the helicase-null cells exhibited HU resistance, we speculated that these cells might also accumulate less DNA breakage following replication arrest. Using PFGE analysis we found that the helicase-null cells indeed showed significantly less DNA breakage ( Fig. 3d ), in line with the findings in human FBH1-depleted cells. 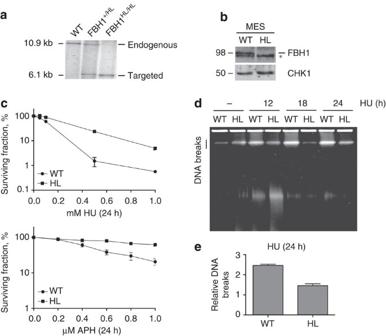Figure 3: Aberrant response to replication stress in murine ES cells devoid of FBH1 helicase activity. (a) Southern blot analysis of targetedFBH1alleles in murine ES cells. Genomic DNA was digested withEcoRI, separated by agarose gel electrophoresis and hybridized with radiolabelled 3′ probe (see Methods). Sizes of the DNA bands are shown to the left. (b) MES cells, either FBH1 wild-type (WT) or helicase-null (HL) were subjected to immunoblotting with the indicated antibodies. The asterisk denotes a cross-reacting species. The sizes of molecular mass standards (in kDa) are shown on the left. (c) MES cells, either FBH1 wild-type (WT) or helicase-null (HL) were left untreated or treated with the indicated doses of HU (Upper) or APH (lower) for 24 h. Cells were plated and surviving clones were scored 10–12 days later. Graph depicting the surviving fractions is shown. Experiments were done in triplicate and error bars represent s.d. (d) MES cells, either FBH1 wild-type (WT) or helicase-null (HL) were left untreated or treated with HU (1 mM) for the indicated timepoints. Cells were collected and subjected to PFGE analysis. Bands representing DNA breaks are shown. (e) Quantification of (d). Experiments were done in triplicates for the 24 h timepoint, bands were quantified using ImageJ software and error bars represent s.d. Figure 3: Aberrant response to replication stress in murine ES cells devoid of FBH1 helicase activity. ( a ) Southern blot analysis of targeted FBH1 alleles in murine ES cells. Genomic DNA was digested with Eco RI, separated by agarose gel electrophoresis and hybridized with radiolabelled 3′ probe (see Methods). Sizes of the DNA bands are shown to the left. ( b ) MES cells, either FBH1 wild-type (WT) or helicase-null (HL) were subjected to immunoblotting with the indicated antibodies. The asterisk denotes a cross-reacting species. The sizes of molecular mass standards (in kDa) are shown on the left. ( c ) MES cells, either FBH1 wild-type (WT) or helicase-null (HL) were left untreated or treated with the indicated doses of HU (Upper) or APH (lower) for 24 h. Cells were plated and surviving clones were scored 10–12 days later. Graph depicting the surviving fractions is shown. Experiments were done in triplicate and error bars represent s.d. ( d ) MES cells, either FBH1 wild-type (WT) or helicase-null (HL) were left untreated or treated with HU (1 mM) for the indicated timepoints. Cells were collected and subjected to PFGE analysis. Bands representing DNA breaks are shown. ( e ) Quantification of ( d ). Experiments were done in triplicates for the 24 h timepoint, bands were quantified using ImageJ software and error bars represent s.d. Full size image FBH1 and MUS81 operate in a common pathway Prolonged HU treatment leads to the collapse of stalled replication forks accompanied by DNA breakage mediated by the MUS81 endonuclease [6] . Ablation of MUS81, therefore, prevents the accumulation of DSBs following HU treatment. To test if prevention of MUS81-specific DNA breakage would have any impact on DNA DSB formation and survival after HU, we depleted MUS81 using siRNA ( Fig. 4a , and Supplementary Fig. S3 ). Similar to FBH1 depletion, MUS81-depleted cells also exhibited increased resistance to HU treatment ( Fig. 4b , and Supplementary Fig. S3B ). In line with this, we also found that depletion of the MUS81 co-factor EME1 made cells significantly more resistant to HU treatment ( Supplementary Fig. S3 ). Moreover, depletion of SLX4 (an important MUS81 regulatory factor) resulted in a marked decrease in DNA breakage following HU treatment (data not shown). Interestingly, the combined depletion of MUS81 and FBH1 did not have any additional effect on HU survival, suggesting that they operate in the same pathway ( Fig. 4b ). To corroborate this, we used PFGE to detect DNA DSB formation. As expected, cells individually depleted for MUS81 and FBH1 showed a strong reduction in DNA breaks following prolonged HU treatment ( Fig. 4c ), whereas no significant additional effect was observed upon co-depletion. To further test the possibility that FBH1 and MUS81 might operate in the same pathway, we carried out clonogenic survival assays of cells overexpressing FBH1 in a mock or MUS81-depleted background ( Fig. 4d ). Interestingly, depletion of MUS81 rescued the FBH1-induced cell death ( Fig. 4e ), arguing that these two factors operate in the same pathway and that FBH1 operates upstream of MUS81. Taken together, our data indicate that FBH1 and MUS81 operate in a common pathway in the cellular response to replication stress ( Fig. 4f ). 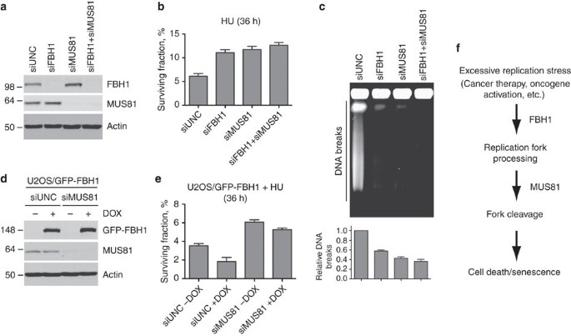Figure 4: FBH1 and MUS81 operate in a common pathway in response to replication stress. (a) U2OS cells were transfected with the indicated siRNAs for 48 h. Cells were collected and subjected to immunoblotting with the indicated antibodies. The sizes of molecular mass standards (in kDa) are shown on the left. (b) U2OS cells were transfected with the indicated siRNAs for 48 h before treatment with 2 mM HU for 36 h. Cells were plated and surviving clones were scored 10–12 days later. Bar chart depicting the surviving fractions is shown. Experiments were done in triplicate and error bars represent s.d. (c) U2OS cells were transfected with the indicated siRNAs for 48 h before treatment with 2 mM HU for 36 h. Cells were collected and subjected to PFGE analysis. Bands representing DNA breaks are shown. (Bottom) Experiments were done in triplicate, bands were quantified using ImageJ software and error bars represent s.d. (d) Immunoblotting analysis of samples from (e). The sizes of molecular mass standards (in kDa) are shown on the left. (e) U2OS/GFP-FBH1 WT cells were transfected with negative control or MUS81 siRNA for 24 h, followed by induction with doxycycline or not for another 24 h. Cells were plated before treatment with 2 mM HU for 36 h and surviving clones were scored 10–12 days later. Bar chart depicting the surviving fractions is shown. Experiments were done in triplicate and error bars represent s.d. (f) Model depicting how FBH1 can promote fork cleavage and cell death after replication stress. HU treatment induces replication arrest and whereby FBH1 remodels the fork to initiate checkpoint signalling. The remodelled fork also facilitates cleavage by MUS81, which promotes cell death. Figure 4: FBH1 and MUS81 operate in a common pathway in response to replication stress. ( a ) U2OS cells were transfected with the indicated siRNAs for 48 h. Cells were collected and subjected to immunoblotting with the indicated antibodies. The sizes of molecular mass standards (in kDa) are shown on the left. ( b ) U2OS cells were transfected with the indicated siRNAs for 48 h before treatment with 2 mM HU for 36 h. Cells were plated and surviving clones were scored 10–12 days later. Bar chart depicting the surviving fractions is shown. Experiments were done in triplicate and error bars represent s.d. ( c ) U2OS cells were transfected with the indicated siRNAs for 48 h before treatment with 2 mM HU for 36 h. Cells were collected and subjected to PFGE analysis. Bands representing DNA breaks are shown. (Bottom) Experiments were done in triplicate, bands were quantified using ImageJ software and error bars represent s.d. ( d ) Immunoblotting analysis of samples from ( e ). The sizes of molecular mass standards (in kDa) are shown on the left. ( e ) U2OS/GFP-FBH1 WT cells were transfected with negative control or MUS81 siRNA for 24 h, followed by induction with doxycycline or not for another 24 h. Cells were plated before treatment with 2 mM HU for 36 h and surviving clones were scored 10–12 days later. Bar chart depicting the surviving fractions is shown. Experiments were done in triplicate and error bars represent s.d. ( f ) Model depicting how FBH1 can promote fork cleavage and cell death after replication stress. HU treatment induces replication arrest and whereby FBH1 remodels the fork to initiate checkpoint signalling. The remodelled fork also facilitates cleavage by MUS81, which promotes cell death. Full size image Cells encounter replication stress both during unperturbed cell cycles and in situations where nucleotide pools are insufficient, which can be caused by activation of oncogenes or when treated with HU in the clinic [20] . Replication forks that are exposed to replication stress can stall, but nevertheless they seem to retain the capability to restart productive DNA synthesis for a period of time. Eventually, however, stalled forks become irreversably inactivated and collapse, as evidenced by disassembly of the replisome and subsequent generation of DNA DSBs [15] . The mechanisms by which stalled forks are processed and the biological role of this processing are not well understood in mammalian cells. Replication arrest does not induce detectable numbers of DNA DSBs at early times after treatment, but these breaks do arise at later stages induced by HU or aphidicolin (around 18–24 h after treatment) [15] , where the fork is subjected to cleavage by the MUS81 endonuclease [6] . Our data have uncovered a critical role for FBH1 in MUS81-induced cleavage of stalled replication forks, as DSBs were not detected in FBH1-depleted cells following HU treatment. These nucleolytic events were found to be fully dependent on the helicase activity of FBH1. Interestingly, FBH1 is a UvrD-type helicase, which preferentially unwinds dsDNA with a protruding ssDNA tail of at least 18 nucleotides, a substrate mostly seen in stalled replication forks. Like UvrD, FBH1 displays 3′–5′ directionality for its unwinding activity [10] . In relation to a stalled fork, this would allow unwinding of the lagging strand, potentially generating a substrate for MUS81. However, the precise substrate recognized by MUS81 at the fork is not known, but possibilities include Holliday junctions generated by replication fork regression or the stalled fork itself [8] , [21] , [22] . Our data on the role of MUS81 in the response to HU are in agreement with Hanada et al. [6] with regard to MUS81-induced DNA DSB formation. Yet, Hanada et al. [6] found that genetic ablation of MUS81 led to HU-sensitivity. Owing to the transient nature of the siRNA experiments performed in this study, MUS81 and EME1 proteins are absent during the DNA DSB formation, but the proteins will eventually reappear during the clonogenic survival assay where they can contribute to important cellular functions such as DNA repair and DNA replication, thereby supporting survival. However, genetic ablation does not allow proteins to reappear, and the complete absence of MUS81 and EME1 is likely responsible for the poor survival following excess replication stress. The functional role of fork cleavage in the cellular response to replication stress is still uncertain. However, the DBSs could potentially participate in replication fork restart, but notably, MUS81 has a minor role in fork restart in human cells, because the majority of forks are thought to be inactive when cleaved [7] . In line with this, forks might not necessarily need to restart because replication can be completed from neighbouring origins [23] . Once a replication fork from an adjacent origin reaches an unrepaired collapsed fork, this would result in a two-ended DSB that can undergo repair via HR or nonhomologous end-joining. Our data suggest that FBH1- and MUS81-mediated DNA DSBs following prolonged replication stress trigger strong checkpoint signalling and cell death. We observed that although fork processing is aberrant in the absence of FBH1, cells were able to resist the lethal effects of replication stress better. Importantly, the function of FBH1 is specific for DNA breakage following replication stress, as FBH1 function does participate in DSB formation by other means. It seems very likely that the increased replication stress tolerance may relate to the reduction in DNA DSBs, which lowers checkpoint and pro-apoptotic responses allowing the enhanced recovery of cells. Hence, although intuitively one might imagine that cells would be better off without FBH1, we suggest that FBH1-driven fork collapse both protects the genome on the cellular level as well as the organism in the long run by eliminating unstable cells with potentially pre-neoplastic genetic abnormalities. On that note, as replication stress also occurs during oncogene activation [4] , our data imply that FBH1 can have an important role in the response to oncogene activation, where FBH1 might also help eliminate cells with replicative stress and suppress the generation of pathological genetic changes. Our data support the hypothesis that FBH1 controls a mechanism to eliminate cells via apoptosis under conditions of elevated replication stress (and oncogene activation) when too many forks have collapsed and restart efforts can be harmful in allowing the propagation of cells with genomic instability. Our results also have clinical relevance in providing insight into the response to genotoxic stress caused by HU, a chemotherapeutic drug used in the treatment of a number of malignancies, as well as polycythemia vera and sickle cell anemia [24] , [25] . Indeed, several DNA replication inhibitors, including gemcitabine, 6-thioguanine and Fludarabine phosphate, are used for the treatment of a number of a wide range of cancers [24] . Finally, our findings suggest that the assessment of FBH1 functional status might potentially be used to identify patients that would benefit from treatment with HU or other drugs with a similar mechanism of action. Cells, chemicals, and siRNA The U2OS cell lines were grown in Dulbecco’s modified Eagle’s medium (DMEM) with 10% fetal bovine serum . Generation of U2OS cell lines carrying inducible expression vectors of GFP-FBH1 WT and helicase dead (D698N) were described previously [9] . The following drugs were used in this study: HU, camptothecin, aphidicolin, nocodazole and mirin (Sigma), ATM inhibitor (KU55933, Tocris Bioscience). Ionizing radiation was administered using a X-ray apparatus (Faxitron). For siRNA transfections, Lipofectamine RNAiMAX (Invitrogen) was used according to the manufacturer’s instructions, with the modification that the transfection reagent was removed 4–6 h after addition, and fresh media added. The siRNA sequences used for knockdown are (5′–3′): FBH1#1 (GGGAUGUUCUUUUGAUAAA), FBH1#2 (AAACAAAACCUCGUCAUUA), MUS81 (CAGCCCUGGUGGAUCGAUA), MUS81#2 (GGGCAUUGCAGCUUGGAAU), EME1#1 (CAGACAUAGCUGAAACUGU), and  EME1#2 (GGAUAAAGAACGCCAGAAU). A pool of the individual FBH1 siRNAs was used for depletion experiments where indicated ( Supplementary Fig. S1 ). Generation of FBH1 helicase-null MES cells Two targeting vectors for a mutant FBH1 gene containing deletion of helicase domains II and III and either a puromycin or neomycin resistant gene plus an HSV domain were introduced into R1 mouse ES cells [25] by electroporation ( Supplementary Fig. S2 ). To confirm the gene targeting on the 5′ side of the targeting site, purified genomic DNA was digested with Bam HI and Hind III. The digested DNA was hybridized with the 5′ external probe ( Supplementary Fig. S2 ). To confirm the gene targeting on the 3′ side of the targeting site, purified genomic DNA was digested with Eco RI and using a probe to hybridize to the 3′end ( Fig. 3a ). Culturing of MES Cells Plates for the mouse ES cell culture were coated using 0.1% type-A gelatin (Sigma) for 5 min before used. Mouse ES cells were maintained in 50% buffalo rat liver-conditioned medium/50% fresh DMEM supplemented with 10% fetal calf serum, 0.1% β-mercaptoethanol, 2.4 mM glutamine, 1,000 U ml −1 leukaemia inhibitory factor (Gibco) and non-essential amino acids. Cells were grown at 37 °C in a humidified atmosphere containing 5% CO 2 . Clonogenic survival assays Cells were counted and seeded on plates for 24 h, followed by drug treatment with for the indicated times. After treatment, the cells were washed with PBS and were then grown in fresh medium for 10–12 days. Colonies were fixed, stained with Coomassie solution (0.1% Coomassie Blue, 7% acetic acid, 50% methanol), and counted. All experiments were performed in triplicate. Same procedure was used for mouse ES cells, except they were seeded on gelatinized dishes. Flow cytometry To prepare cells for flow cytometry, U2OS cells were fixed in 70% ethanol. DNA was stained with 0.1 mg ml −1 propidium iodide containing RNase (20 μg ml −1 ) for 30 min at 37 °C. For EdU labelling, cells were incubated with 10 μM EdU for 30 min before harvest. Click-it reaction was performed according to the manufacturers description (Invitrogen). Flow cytometry was performed on a FACS Calibur (BD Biosciences) using CellQuest Pro software (Becton Dickinson). Immunoblotting and antibodies Cells were lyzed on ice in cold EBC-buffer (150 mM NaCl; 50 mM TRIS pH 7.4; 1 mM EDTA; 0.5% NP-40/Igepal) containing protease inhibitors (1% aprotinin, 5 μg ml −1 leupeptin, 1 mM PMSF), phosphatase inhibitors (50 mM NaF; β-glycerophosphate; 0.5 μM Calyculin A) and 1 mM DTT. The lysates were sonicated using a digital sonifier (102C CE Converter; Branson). Proteins were separated by SDS–PAGE and transferred to a nitrocellulose membrane. Blocking and blotting with primary antibodies were performed in PBS-T supplemented with 5% skimmed milk powder. Proteins were visualized on films using secondary HRP-conjugated antibodies (1:10,000; Vector Laboratories) and ECL (GE Healthcare). Films were developed using an x-ray machine (Valsoe; Ferrania Technologies). The following commercial rabbit antibodies were used in this study: phospho-CHK1-S345 (no. 2348, Cell Signalling), phospho-CHK2-T68 (no. 2661, Cell Signalling), CtIP (BL1914, Bethyl Labs), GFP (FL, SCBT), RPA2 S4/8 (A300-245, Bethyl Labs) and p53-S15 (no. 9284, Cell Signalling). The following commercial mouse antibodies were used in this study: CHK1 (DCS-310; SCBT), CHK2 (DCS-270, SCBT), phospho-ATM-S1981 (Rockland), ATM (11G12, Abcam), γH2AX (JBW301, Millipore), RPA (NA19L, Calbiochem), p53 (DO-1, supernatant), MCM7 (DCS-141, ascites), EME1 (7h2/1, ImmuQuest) and MUS81 (MTA30 2G10, Abcam). Rabbit antibodies raised against hFBH1 were described previously [9] . Immunofluorescence Cells were grown on coverslips and fixed in Lillies (4% formaldehyde) with or without prior pre-extraction in CSK buffer (0.5% Triton X-100 in 20 mM Hepes pH 7.4; 50 mM NaCl; 3 mM MgCl 2 ; and 300 mM sucrose), permeabilized in 0.2% Triton X-100/PBS and incubated with the indicated antibodies diluted in DMEM supplemented with 10% serum. Samples were then stained with secondary Alexa Fluor conjugated antibodies and mounted on glass slides using Vectashield mounting medium with DAPI (Vector Laboratories). Pulsed-field gel electrophoresis For directly assessing cellular DNA breaks, 10 6 cells were collected after indicated treatment and casted into agarose inserts (plugs) before incubation in proteinase K buffer (0.5 M EDTA; 1% N -laurylsarcosyl; 1 mg ml −1 proteinase K) at 50 °C for 24 h. Plugs were washed four times in TE buffer (10 mM TRIS; 50 mM EDTA) and loaded onto a 1% agarose gel (pulsed-field grade, Bio-Rad) and separated by PFGE apparatus for 20 h at 120 o angle, 60–240 s switch time, 4 V cm −1 (CHEF DR III, Bio-Rad). For MES cells, the gel was run on a Rotaphor PFGE apparatus (Biometra, Germany). The gel was subsequently stained with ethidium bromide and visualized using Quantity One software (Bio-Rad). Fibre assay DNA fibre assays using U2OS cells were performed essentially as described previously [11] . Reverse transcriptase polymerase chain reaction (RT–PCR) First-strand cDNA was synthesized by incubating 3 μg isolated mRNA, 50 ng random hexamers and 0.25 mM of each deoxynucleotide triphosphate at 65 o C for 5 min. After chilling, reverse transcriptase, dithiothreitol and RNase inhibitor (Invitrogen Superscript III First-Strand Synthesis System for RT–PCR 18080-051) were added, and cDNA synthesis was continued at 20 o C for 10 min followed by 50 o C for 50 min. The reaction was inactivated by the addition of RNase H. PCR reactions were prepared in 50 μl volumes containing 1x thermophilic DNA pol buffer, 2.5 mM MgCl 2 , 100 μM each of dNTP, 0.5 μM of each primer, ~20 ng cDNA and 1 unit of taq DNA polymerase. The primers used were as follows (5′–3′): 5′mFbh1-ex1 (AGTGGTCGACTGCCATCATTTG), 3′revmFbh1-ex2 (AATGTCCTCAATGTCTCGGCCA), 5′mFbh1-ex7 (GAGCCTCTCCAGGTGGTAAAAA), 3′revmFbh1-ex11 (ATGCCTCTTCTTTGCATTCCCC), 5′mFbh1-ex16 (GGGTGCATAAAGAAGGCTTCAG), and  3′revmFbh1-ex19 (CTTCATGGTAAGGATGGTGTCC). How to cite this article: Fugger et al. FBH1 co-operates with MUS81 in inducing DNA double-strand breaks and cell death following replication stress. Nat. Commun. 4:1423 doi: 10.1038/ncomms2395 (2013).